Disrupting malaria parasite AMA1–RON2 interaction with a small molecule prevents erythrocyte invasion Plasmodium falciparum resistance to artemisinin derivatives, the first-line antimalarial drug, drives the search for new classes of chemotherapeutic agents. Current discovery is primarily directed against the intracellular forms of the parasite. However, late schizont-infected red blood cells (RBCs) may still rupture and cause disease by sequestration; consequently targeting invasion may reduce disease severity. Merozoite invasion of RBCs requires interaction between two parasite proteins AMA1 and RON2. Here we identify the first inhibitor of this interaction that also blocks merozoite invasion in genetically distinct parasites by screening a library of over 21,000 compounds. We demonstrate that this inhibition is mediated by the small molecule binding to AMA1 and blocking the formation of AMA1–RON complex. Electron microscopy confirms that the inhibitor prevents junction formation, a critical step in invasion that results from AMA1–RON2 binding. This study uncovers a strategy that will allow for highly effective combination therapies alongside existing antimalarial drugs. P lasmodium falciparum ( Pf ) infects over 300 million people worldwide causing more than 1 million deaths annually, mostly in young children and pregnant women [1] . Currently there is no vaccine available, and there is widespread resistance to common antimalarial drugs [2] . Recent data suggest the emergence of resistance against artemisinin derivatives, the current first-line defence against malaria [3] , [4] . This warrants novel, alternative approaches for developing new therapeutics. Clinical manifestation of the disease is due to the intraerythrocytic forms of the parasite (see (ref. 5 ) for a review of malaria biology and disease pathogenesis), which on maturation to the schizont stage release merozoites, the invasive form of Pf . Invasion is a rapid process that begins with an initial weak attachment of the merozoites to the RBC, followed by reorientation that brings the apical end of the merozoite into close apposition with the RBC surface [6] , [7] . The commitment of merozoites to invade RBCs is marked by the formation of a firm junction between the apically oriented merozoite and the RBC [7] . Every RBC that is invaded produces 16–32 new merozoites. Invaded RBCs can sequester despite treatment [8] . Therefore, targeting invasion will be a critical component for the development of successful antimalarial therapies. However, existing antimalarial drugs primarily target the intracellular stage of the developing parasites. The potential targets for drug development against merozoite invasion and release have recently been reviewed [5] . Protein–protein interactions (PPIs) have crucial roles in numerous biological processes including disease pathology and host–pathogen interactions. Relatively small regions of the interface of PPIs, so-called ‘hot-spots’, can provide exquisite specificity, and are essential for high-affinity binding [9] , [10] . Hence these orthosteric sites (ligand-binding sites) are attractive targets for small-molecule PPI inhibitors as they allow for interfering with them in a highly specific manner. For instance, Nutlin3, a small-molecule PPI inhibitor of MDM2–p53 interaction [11] that reactivates p53 function is now in clinical trials to treat cancer [12] , [13] . Furthermore, small-molecule inhibitors of PPIs involved in successful viral entry into host cells such as HIV gp120-CCR5 chemokine receptor [14] , dengue virus envelope protein E trimerization that mediates membrane fusion [15] and ebola virus glycoprotein-host Niemann-Pick C1 protein [16] have been identified. Hence small-molecule PPI inhibitors offer attractive opportunities to target host–parasite interactions and prevent disease. One such essential PPI is between two parasite proteins, apical membrane antigen 1 (AMA1), which is translocated on to the merozoite surface, and rhoptry neck protein 2 (RON2), which is transferred to the RBC membrane during invasion [17] , [18] , [19] . We have recently shown that the interaction between AMA1 and RON2 is essential for junction formation with the RBC [19] , an irreversible step that commits the parasite to invasion. A short RON2 peptide (RON2L) that binds to a hydrophobic pocket on AMA1 is sufficient to compete with the native RON2 protein and inhibit invasion [19] , [20] . Two intimately associated PAN domains in AMA1 form a highly conserved hydrophobic pocket [21] . The binding of the RON2 peptide to the hydrophobic pocket in AMA1 [22] is required to trigger the formation of the moving junction [19] . The junction provides a firm anchor for the parasite to pull itself into the RBC using its actin–myosin motor. Unlike the other steps in invasion that use functionally redundant proteins, there is only one AMA1 and RON2 in Plasmodium , and there are no alternative pathways. Moreover, the region corresponding to RON2 peptide and the key residues in the AMA1 hydrophobic pocket, including Phe183 that is required for RON2 binding [22] , is conserved among all Pf isolates. This indicates a functional constraint governing an essential step in invasion and represents a novel target that can potentially be exploited for antimalarial therapy. Here we present results identifying small-molecule inhibitors of AMA1–RON2 interaction that block merozoite invasion of RBCs. We show that the inhibitor binds to AMA1 and prevents its interaction with RON2. In doing so, it disrupts the function of AMA1–RON2 interaction, namely, junction formation, a crucial step in merozoite invasion of RBCs. Such inhibitors of merozoite invasion used in combination with existing antimalarials hold great promise as a novel therapeutic approach in the fight against malaria. Screen for the assessment of AMA1–RON2 interaction A short RON2 peptide (RON2L) corresponding to the binding region on AMA1 is sufficient to compete with the native RON2 protein and inhibit merozoite invasion of RBCs [19] , [20] . We developed a quantitative high-throughput screen (HTS) using the AlphaScreen technology ( Fig. 1a ) to investigate the interaction between AMA1 and RON2L. In this assay, streptavidin-coated donor beads bind to the biotinylated RON2L peptide, whereas the nickel chelate acceptor beads bind to the His-tagged AMA1 recombinant protein. Interaction between RON2L and AMA1 brings the donor and acceptor beads into close proximity. Upon excitation at 680 nm, the donor beads containing the photosensitizer phthalocyanine convert ambient oxygen to singlet oxygen (4 μs half-life). The close proximity of RON2 and AMA1 allows for the diffusion and efficient transfer of energy from the singlet oxygen to thioxene derivatives within the acceptor bead, which emits light in the 520–620 nm region. This proximity-dependent transfer of energy and the homogenous detection of protein–protein interactions allow for a highly sensitive high-throughput screen. Disruption of AMA1–RON2L interaction by small-molecule inhibitors will result in reduced or no emission signal depending on the strength of the inhibition. 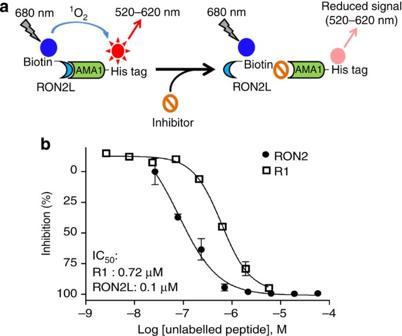Figure 1: Quantitative high-throughput assay to identify inhibitors of the AMA1–RON2 interaction. (a) In the AlphaScreen assay, streptavidin-coated donor beads captures biotin-tagged RON2L peptide and the nickel-coated acceptor beads binds to His-tagged AMA1(3D7 allele). In the absence of inhibitor, excitation of the donor beads at 680 nm results in the production of singlet oxygen, followed by short-distance diffusion (<200 nm) and energy transfer to the acceptor beads, in turn resulting in emission at 520–620 nm. Disruption of the interaction leads to reduced or no signal. (b) R1 peptide that specifically binds 3D7 allele of AMA1 (square) and the unlabelled RON2L peptide (black circle) were used as positive controls for inhibitors in the AlphaScreen assay. Error bars show±s.e.m. from two independent experiments. Figure 1: Quantitative high-throughput assay to identify inhibitors of the AMA1–RON2 interaction. ( a ) In the AlphaScreen assay, streptavidin-coated donor beads captures biotin-tagged RON2L peptide and the nickel-coated acceptor beads binds to His-tagged AMA1(3D7 allele). In the absence of inhibitor, excitation of the donor beads at 680 nm results in the production of singlet oxygen, followed by short-distance diffusion (<200 nm) and energy transfer to the acceptor beads, in turn resulting in emission at 520–620 nm. Disruption of the interaction leads to reduced or no signal. ( b ) R1 peptide that specifically binds 3D7 allele of AMA1 (square) and the unlabelled RON2L peptide (black circle) were used as positive controls for inhibitors in the AlphaScreen assay. Error bars show±s.e.m. from two independent experiments. Full size image The HTS assay was miniaturized and optimized in a 1,536-well plate format. The assay displayed minimal well-to-well variation and a Z ′ factor [23] of 0.7 or greater ( Supplementary Fig. S1 ), indicating a robust screen. As there is no known small-molecule inhibitor of the AMA1–RON2 interaction, we validated our screen using the R1 peptide that binds to only AMA1 from the P. falciparum 3D7 clone [24] . The unlabelled R1 peptide exhibited a concentration-dependent inhibition with an IC 50 value of ~0.7 μM ( Fig. 1b ). A second validation was performed using untagged RON2L that competes with biotin-tagged RON2L for binding AMA1 with an IC 50 value of ~0.1 μM ( Fig. 1b ). Screen for small-molecule inhibitors of AMA1–RON2 interaction A pilot screen of 21,733 compounds ( Supplementary Fig. S2 ) was performed at a five-concentration dilution series (92 nM to 114 μM) titration using the AMA1–RON2 AlphaScreen assay. Compounds that showed inhibitory activity in the primary screen were re-screened from fresh stocks in the AlphaScreen assay. False positives may represent compounds that quench singlet oxygen or luminescence signal, or ones that interfere with biotin or nickel chelator beads binding to the affinity tags on RON2 peptide and AMA1. To remove such compounds, we used a counterscreen to measure the binding of AlphaScreen beads to a biotinylated-(His) 6 linker, an analyte serving to bind both donor and acceptor beads outside the context of the AMA1–RON2 interaction. With this approach we confirmed 20 compounds as true hits and 14 of these, chosen based on availability, were used in the downstream assays ( Supplementary Tables S1 and S2 ). AMA1–RON2 inhibitors block merozoite invasion As the AlphaScreen assay used AMA1 corresponding to the 3D7 allele, we tested the compounds using a modified-HTS parasite growth inhibition assay [25] using a heterologous parasite clone (FVO). Seven compounds showed growth inhibition (28–34 μM) in this assay ( Supplementary Table S1 ). As this assay takes over 36 h, some compounds may also affect intraerythrocytic development and cannot be distinguished from the ones that block invasion. To address whether the AMA1–RON2 inhibitors block parasite invasion, we used purified merozoites from a Pf line adapted to retain invasiveness [19] . As merozoite invasion is a very rapid process and takes less than a minute to complete entry into RBCs, this assay allows for unequivocal identification of compounds that block invasion. Purified merozoites were allowed to invade fresh RBCs in the presence of varying concentrations (25 and 50 μM) of the compounds. The efficiency of the compounds to inhibit invasion was measured by counting the number of newly invaded rings. Three compounds, NCGC00015280, NCGC00014044 and NCGC00181034 that block the binding of AMA1 to RON2 ( Table 1 ) also inhibited merozoite invasion ( Fig. 2a and Supplementary Table S1 ). Table 1 Chemical structures and AlphaScreen IC 50 values of three compounds that inhibit AMA1–RON2 interaction and block merozoite invasion from schizont-infected RBCs. 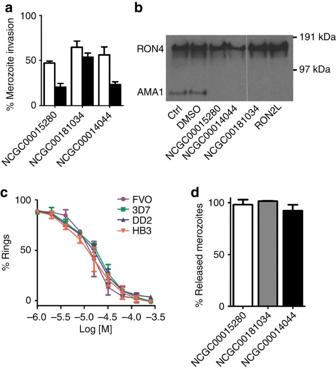Figure 2: Small molecules block AMA1–RON complex formation and inhibit merozoite invasion. (a) Purified merozoites were used to test the effect of the three compounds on invasion of RBCs at 25 μM (white bars) and 50 μM (black bars) for 4 h. Error bars show±s.e.m. from five experiments for NCGC00015280, NCGC00181034 and two for NCGC00014044. (b) Immunoprecipitation assay testing the ability of the inhibitors to block parasite AMA1–RON complex formation. Each inhibitor was used at 100 μM concentration and was immunoprecipitated using anti-RON4 antibody. RON2L peptide was used as a positive control. DMSO (1%), the solvent for the inhibitors, was used as a negative control. Experiments were performed twice and a representative western blot data is shown. (c) NCGC00015280 inhibits merozoite invasion of genetically distinct parasite clones. Purified schizonts from four different parasite clones were allowed to rupture and invade new RBCs for 4–6 h in the presence of varying concentrations of the inhibitor. The number of newly invaded rings was measured by flow cytometry of SYBR green-labelled parasites. IC50: 12 μM (FVO), 14 μM (3D7), 13 μM (DD2) and 10 μM (HB3). Error bars show±s.e.m. from two experiments for each parasite clone. (d) Merozoite release from schizont-infected RBCs is not affected. The effect of the inhibitors on merozoite release was tested at 30 μM, the IC50for invasion. Error bars represent±s.e.m. from three experiments for NCGC00015280, NCGC00181034 and two for NCGC00014044. The number of parasites in the absence of inhibitor was considered 100%. Full size table Figure 2: Small molecules block AMA1–RON complex formation and inhibit merozoite invasion. ( a ) Purified merozoites were used to test the effect of the three compounds on invasion of RBCs at 25 μM (white bars) and 50 μM (black bars) for 4 h. Error bars show±s.e.m. from five experiments for NCGC00015280, NCGC00181034 and two for NCGC00014044. ( b ) Immunoprecipitation assay testing the ability of the inhibitors to block parasite AMA1–RON complex formation. Each inhibitor was used at 100 μM concentration and was immunoprecipitated using anti-RON4 antibody. RON2L peptide was used as a positive control. DMSO (1%), the solvent for the inhibitors, was used as a negative control. Experiments were performed twice and a representative western blot data is shown. ( c ) NCGC00015280 inhibits merozoite invasion of genetically distinct parasite clones. Purified schizonts from four different parasite clones were allowed to rupture and invade new RBCs for 4–6 h in the presence of varying concentrations of the inhibitor. The number of newly invaded rings was measured by flow cytometry of SYBR green-labelled parasites. IC 50 : 12 μM (FVO), 14 μM (3D7), 13 μM (DD2) and 10 μM (HB3). Error bars show±s.e.m. from two experiments for each parasite clone. ( d ) Merozoite release from schizont-infected RBCs is not affected. The effect of the inhibitors on merozoite release was tested at 30 μM, the IC 50 for invasion. Error bars represent±s.e.m. from three experiments for NCGC00015280, NCGC00181034 and two for NCGC00014044. The number of parasites in the absence of inhibitor was considered 100%. Full size image Invasion inhibitors block parasite AMA1–RON complex As the small molecules block merozoite invasion, we tested if they also blocked parasite-derived AMA1–RON2 interaction. Towards this we performed immunoprecipitation of the AMA1–RON complex [26] from schizont-infected RBCs. The RON complex is comprised of rhoptry neck proteins RON2, RON4 and RON5 [18] , [26] . As expected, in the absence of inhibitors, immunoprecipitation of RON4 pulls down AMA1 from parasite extracts ( Fig. 2b ). However, complex formation is disrupted in the presence of AMA1–RON2 inhibitors ( Fig. 2b ). This indicates that the inhibitors block the formation of AMA1–RON2 complex and prevent merozoite invasion of RBCs. AMA1–RON2 inhibitors are strain-transcending AMA1 is highly polymorphic and antibodies against the protein from one parasite clone do not inhibit heterologous clones [27] , [28] . However, the key residues in the AMA1 hydrophobic pocket that bind to RON2, and the region corresponding to RON2L that binds to AMA1 is conserved in all Pf clones. We designed a flow cytometry-based invasion assay to test the ability of the AMA1–RON2 inhibitors to block merozoite invasion of genetically distinct Pf clones. Mature schizont-infected RBCs were allowed to rupture and release merozoites that invade fresh RBCs for 4 h in the presence of different concentrations of the inhibitors. All three compounds were able to block invasion of the four genetically distinct Pf clones (IC 50 : 10–14 μM), including the drug-resistant DD2 clone ( Fig. 2c ) with minimal to no effect on schizont rupture ( Fig. 2d ). Proof-of-concept optimization of an AMA1–RON2 inhibitor First, to rule out the effect of any impurities present in the original compound, we re-synthesized and purified NCGC00015280 to test in our biological assays (see Supplementary Methods ). The re-synthesized compound showed activity similar to that of the original sample confirming NCGC00015280 as an AMA1–RON2 inhibitor that blocks merozoite invasion ( Supplementary Fig. S3 ). Next, we attempted to improve the activity of NCGC00015280 through the synthesis of related analogues, and tested them for invasion inhibition using mature schizonts. Two analogues, NCGC00262650 and NCGC00262654 (see Supplementary Methods ) showed improved inhibition over the parent compound ( Figs 3a,b ). Invasion assay using purified merozoites showed that these two compounds blocked entry of merozoites into RBCs at threefold (9.8 μM) and fivefold (6 μM) lower IC 50 than the parent compound (30 μM), respectively ( Fig. 3c ). At the same concentrations, intracellular growth and merozoite rupture from schizonts were not affected ( Supplementary Fig. S4 ). 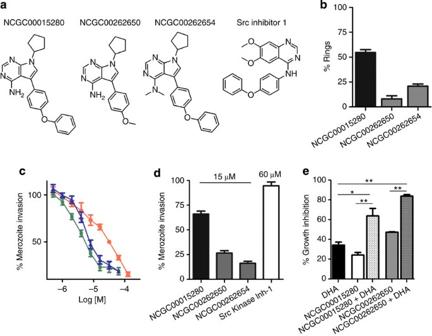Figure 3: Improved efficiency of analogues in blocking merozoite invasion. (a) Structure of two analogues that showed improved potency. (b) Schizont-infected RBCs were allowed to rupture and invade new red cells for 4 h in the presence of 15 μM of the parent compound (black bar) or the two analogues (gray bars). The number of newly invaded rings was measured by flow cytometry. The number of parasites in the absence of inhibitor was considered 100%. Error bars represent±s.e.m. from four independent experiments for each compound. (c) Purified invasive merozoites were allowed to invade RBCs and develop for 3–4 h in the presence of varying concentrations of the two analogues (green and blue lines) and the parent compound (orange line). Invasion efficiency was measured by counting the number of newly formed rings. A three- to fivefold lower IC50(6 and 9.8 μM, respectively) is seen for the two analogues compared with the parent compound (IC50: 30 μM). orange, NCGC00015280; blue, NCGC00262650 and green, NCGC00262654. Error bars represent±s.e.m. from three independent experiments for each compound. (d) Merozoite invasion is not inhibited by a Src Kinase Inhibitor-1, but is blocked by AMA1–RON2 inhibitors. The concentrations of the compounds used are shown in the figure. Error bars represent±s.e.m. from at least two experiments for each compound. The number of parasites in the absence of inhibitor was considered 100%. (e) DHA in combination with invasion inhibitors is more efficient than by itself. Inhibitors NCGC00015280 (8 μM), NCGC00262650 (8 μM) and DHA (3 nM) alone or in combination were tested for growth inhibition. Parasite growth in the absence of any inhibitor was used as a control for no inhibition. Data represents the mean±s.e.m. of 3D7 and FVO parasites performed in duplicates.Pvalues were calculated using one-way analysis of variance and Bonferroni’s post test was performed to compare the effect of the combination treatment over the respective individual compounds. **P<0.01. Figure 3: Improved efficiency of analogues in blocking merozoite invasion. ( a ) Structure of two analogues that showed improved potency. ( b ) Schizont-infected RBCs were allowed to rupture and invade new red cells for 4 h in the presence of 15 μM of the parent compound (black bar) or the two analogues (gray bars). The number of newly invaded rings was measured by flow cytometry. The number of parasites in the absence of inhibitor was considered 100%. Error bars represent±s.e.m. from four independent experiments for each compound. ( c ) Purified invasive merozoites were allowed to invade RBCs and develop for 3–4 h in the presence of varying concentrations of the two analogues (green and blue lines) and the parent compound (orange line). Invasion efficiency was measured by counting the number of newly formed rings. A three- to fivefold lower IC 50 (6 and 9.8 μM, respectively) is seen for the two analogues compared with the parent compound (IC 50 : 30 μM). orange, NCGC00015280; blue, NCGC00262650 and green, NCGC00262654. Error bars represent±s.e.m. from three independent experiments for each compound. ( d ) Merozoite invasion is not inhibited by a Src Kinase Inhibitor-1, but is blocked by AMA1–RON2 inhibitors. The concentrations of the compounds used are shown in the figure. Error bars represent±s.e.m. from at least two experiments for each compound. The number of parasites in the absence of inhibitor was considered 100%. ( e ) DHA in combination with invasion inhibitors is more efficient than by itself. Inhibitors NCGC00015280 (8 μM), NCGC00262650 (8 μM) and DHA (3 nM) alone or in combination were tested for growth inhibition. Parasite growth in the absence of any inhibitor was used as a control for no inhibition. Data represents the mean±s.e.m. of 3D7 and FVO parasites performed in duplicates. P values were calculated using one-way analysis of variance and Bonferroni’s post test was performed to compare the effect of the combination treatment over the respective individual compounds. ** P <0.01. Full size image Merozoite invasion is not affected by Src kinase inhibitors The AMA1–RON2 inhibitor NCGC00015280 was originally identified as a specific Src-family tyrosine kinase inhibitor [29] . However, there are no tyrosine kinases identified in the Plasmodium genome [30] despite the presence of tyrosine-phosphorylated proteins [31] , making it unlikely that the inhibition was due to its effect on a parasite tyrosine kinase. Furthermore, we used another Src kinase inhibitor I [32] to examine the possibility of a Src kinase-like enzyme that may function during merozoite invasion. Although the parent compound and the two analogues show potent inhibition, the unrelated Src kinase inhibitor I (IC 50 : 44–88 nM) does not block merozoite invasion even at 60 μM ( Fig. 3d ). This suggests that the small-molecule inhibitor blocks merozoite invasion by preventing the formation of the AMA1–RON2 complex. Invasion inhibitors in combination with artemisinin There is increasing evidence for the development of resistance against the first-line antimalarial artemisinin [3] , [4] and existing partner drugs [2] . Therefore, we tested the usefulness of merozoite invasion inhibitors NCGC00015280 and NCGC00262650 in combination with dihydroartemisinin (DHA), the active metabolite. Synchronized schizonts (3D7 and FVO clones) were allowed to rupture, invade in the presence of either individual compounds or in combination, and allowed to develop within RBCs for 72 h. Indeed, the efficiency of growth inhibition is enhanced when both the intracellular parasites and merozoite invasion were simultaneously targeted ( Fig. 3e ). Such combinations offer a promising approach to prevent, as well as, treat artemisinin-resistant parasites. PPI inhibitor blocks merozoite invasion by binding to AMA1 Small molecules identified through our HTS assay may exert their inhibition by binding to either AMA1 or RON2, even though the probable orthosteric hot-spot may lie in the hydrophobic grove of AMA1. To address the mode of inhibition, we performed a depletion assay to assess the binding of the small molecule NCGC00262650 to either his-tagged recombinant AMA1 protein or biotin-tagged RON2L peptide. The ability of AMA1 or RON2L to bind to the inhibitor was assessed by performing invasion assays using inhibitor-depleted supernatants. Recombinant AMA1 was very effective in depleting the inhibitory activity; however RON2L was not ( Fig. 4a ). Significantly, recombinant proteins representing two diverse alleles of AMA1 from the 3D7 and FVO parasites bound to the compound and depleted inhibitory activity( Fig. 4a ). This clearly demonstrates that the mode of action of the small molecule is mediated through the binding of AMA1 and blocking its interaction with RON2. Furthermore, SPR experiments also confirmed the binding of the small-molecule inhibitors to AMA1 ( Supplementary Fig. S7 ), though the affinity could not be determined due to poor solubility (precipitation) of the inhibitors in the SPR buffer. We also performed a qualitative immunofluorescence assay using fluorescein isothiocyanate (FITC)-labelled RON2 peptide to evaluate the binding of RON2 to parasite AMA1 ( Fig. 4b ). This assay was previously used to demonstrate the binding of RON2 peptide to AMA1 present in the micronemes [33] . Although FITC-labelled PfRON2L binds to schizonts, binding is prevented in the presence of the inhibitor ( Fig. 4b ). 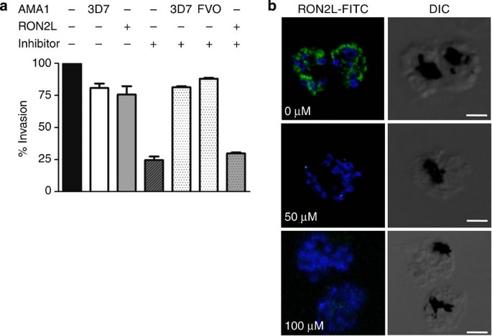Figure 4: Mode of action of the inhibitor NCGC00262650 is mediated through binding of AMA1. (a) The mode of inhibition of the small molecule was studied by a depletion assay using either his-tagged recombinant AMA1 or biotin-tagged RON2L peptide. The ability of AMA1 or RON2 to bind the inhibitor was assessed by performing invasion assays using inhibitor-depleted supernatants. Five-hundred picomoles of either recombinant AMA1 (both 3D7 and FVO allele) or RON2L peptide bound to magnetic beads was used to deplete 500 pmol of the inhibitor (final concentration 10 μM). Error bars represent±s.e.m. from two experiments. (b) Immunofluorescence assay using FITC-labelled RON2L peptide. FITC-labelled RON2 peptide binds to AMA1 in the mature schizonts in the absence of inhibitors, whereas pre-incubation with inhibitor NCGC00015280 prevents binding of the peptide. Similar results were obtained with the analogue NCGC00262650 and the inhibitor NCGC00181034 (data not shown). Scale bars, 3 μM. Figure 4: Mode of action of the inhibitor NCGC00262650 is mediated through binding of AMA1. ( a ) The mode of inhibition of the small molecule was studied by a depletion assay using either his-tagged recombinant AMA1 or biotin-tagged RON2L peptide. The ability of AMA1 or RON2 to bind the inhibitor was assessed by performing invasion assays using inhibitor-depleted supernatants. Five-hundred picomoles of either recombinant AMA1 (both 3D7 and FVO allele) or RON2L peptide bound to magnetic beads was used to deplete 500 pmol of the inhibitor (final concentration 10 μM). Error bars represent±s.e.m. from two experiments. ( b ) Immunofluorescence assay using FITC-labelled RON2L peptide. FITC-labelled RON2 peptide binds to AMA1 in the mature schizonts in the absence of inhibitors, whereas pre-incubation with inhibitor NCGC00015280 prevents binding of the peptide. Similar results were obtained with the analogue NCGC00262650 and the inhibitor NCGC00181034 (data not shown). Scale bars, 3 μM. Full size image AMA1–RON2 inhibitor blocks junction formation We have previously shown that the binding of RON2 to AMA1 triggers junction formation, which commits the merozoite for invasion [19] . As the inhibitors bind to AMA1 and prevent binding of RON2, we performed electron microscopy to determine the precise step at which merozoite invasion was blocked. The actin–myosin motor that propels the merozoite during invasion is constantly active [19] . Hence cytochalasin D (cyto D) that blocks actin polymerization was used to prevent the attached merozoites from falling-off RBCs. In the presence of cyto D alone, merozoites were able to re-orient and form a junction ( Fig. 5 and Supplementary Fig. S5 ). However, in the presence of the inhibitors (NCGC00015280 and NCGC00262650), despite the merozoites being able to attach to RBC and re-orient ( Fig. 5b ), junction formation was severely affected ( Fig. 5c ). 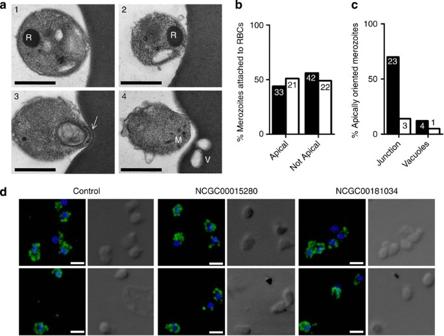Figure 5: AMA1–RON2 inhibitor blocks junction formation. (a) Transmission electron microscopy showing the different stages of RBC invasion in the presence of 2 μM cyto D, namely, attachment (1), reorientation (2), junction formation (3) and rhoptry bulb secretion (4). R: rhoptry, M: micronemes, V: vacuoles; White arrow: junction. Scale bars, 250 nm. (b) The percentage of merozoites that are attached to RBCs in the presence (white bars) or absence (black bars) of the AMA1–RON2 inhibitor NCGC00015280/NCGC00262650. (c) The percentage of apically oriented merozoites in the presence (white bars) or absence (black bars) of the inhibitor that forms a junction and RBCs with vacuoles (indicative of rhoptry bulb secretion). Numbers within each bar represent the number of merozoite-attached RBCs in each category. Data were pooled from two independent experiments without inhibitor and one each with inhibitor NCGC00015280 and NCGC00262650. Scale bars, 250 nm. (d) AMA1 secretion from micronemes is not affected. Merozoites released from schizonts in the absence (control) or presence of inhibitors NCGC00015280 (60 μM) and NCGC00181034 (60 μM) were analysed using polyclonal antibodies to AMA1. Scale bars, 1 μM. Figure 5: AMA1–RON2 inhibitor blocks junction formation. ( a ) Transmission electron microscopy showing the different stages of RBC invasion in the presence of 2 μM cyto D, namely, attachment (1), reorientation (2), junction formation (3) and rhoptry bulb secretion (4). R: rhoptry, M: micronemes, V: vacuoles; White arrow: junction. Scale bars, 250 nm. ( b ) The percentage of merozoites that are attached to RBCs in the presence (white bars) or absence (black bars) of the AMA1–RON2 inhibitor NCGC00015280/NCGC00262650. ( c ) The percentage of apically oriented merozoites in the presence (white bars) or absence (black bars) of the inhibitor that forms a junction and RBCs with vacuoles (indicative of rhoptry bulb secretion). Numbers within each bar represent the number of merozoite-attached RBCs in each category. Data were pooled from two independent experiments without inhibitor and one each with inhibitor NCGC00015280 and NCGC00262650. Scale bars, 250 nm. ( d ) AMA1 secretion from micronemes is not affected. Merozoites released from schizonts in the absence (control) or presence of inhibitors NCGC00015280 (60 μM) and NCGC00181034 (60 μM) were analysed using polyclonal antibodies to AMA1. Scale bars, 1 μM. Full size image On rupture of merozoites from the schizonts, AMA1 is secreted from the micronemes on to the merozoite surface [34] . We tested by immunofluorescence assay under non-permeabilizing conditions, if the binding of the inhibitor (NCGC00015280 and NCGC00181034) to AMA1 before schizont rupture affected its release on to the merozoite surface. Similar AMA1 staining was observed on merozoites that were released in the presence or absence of inhibitors ( Fig. 5d ). Similar data was observed with NCGC00262650 (not shown). These data indicate that processes that regulate microneme release are not affected, and that the inhibitors specifically block AMA1–RON2 interaction and junction formation, thereby inhibiting merozoite invasion of RBCs. Successful proliferation and transmission of pathogens involve critical PPIs during host-cell entry. Targeting such interactions provide an effective way of preventing diseases. Merozoites, the invasive form of the malaria parasite, utilize several unique PPIs to mediate their entry into RBCs. Vaccines targeting these parasite surface receptors have largely been unsuccessful, and are thought to be mainly due to antigenic diversity in the different parasite clones. However, many PPIs involve ‘hot-spots’, relatively small parts of the protein that mediate binding [9] , [10] . These regions tend to be more conserved but may be hidden from the host immune system. Targeting these ‘hot-spots’ by small-molecule inhibitors provides an alternative strategy for defence against pathogens. This study represents the first attempt to develop novel antimalarial compounds based on small-molecule inhibitors of an essential parasite protein–protein interaction required for RBC invasion. We have developed a high-throughput assay to identify small molecules that will block the binding of RON2 to AMA1 and inhibit merozoite invasion of RBCs. The binding of the RON2 peptide to AMA1 triggers junction formation and invasion [19] . The basis of pocket formation is often at the junction of two domains in a protein [35] , which in AMA1 is formed by two PAN apple domains [21] . The RON2 peptide fits snugly into the hydrophobic pocket of AMA1 [22] and, if blocked by small molecules, could lead to powerful new antimalarial drugs. We screened 21,733 small molecules and identified 20 that blocked binding, with IC 50 values between 13 and 29 μM. Importantly, we have used a variety of assays to demonstrate efficacy against multiple Pf clones. The first is a high-throughput assay for molecules that block Pf invasion. Seven were active in a similar range of IC 50 and seven were inactive ( Supplementary Table S1 ). Six were not tested further due to the lack of compound availability. To exclude potential toxicity in the initial test against schizont-infected RBCs, we performed two additional studies. First, the number of released merozoites in a 4-h period was evaluated, as toxicity would suppress parasite growth and merozoite release. Second, the active compounds in the schizont-infected RBC invasion assay were tested with viable merozoites and only three showed good activity. The two biological assays using schizonts or merozoites addressed different questions. In the first, the exposure of schizont-infected RBCs to the drug reflected the way that the drug would be used in humans. If it is inactive in this assay, then the small-molecule inhibitor is not of interest because its accessibility to AMA1 in the parasitized RBC or after merozoite release from the RBC is ineffective. Assays using purified merozoites demonstrate unequivocally the effect of the small molecules to block invasion and not due to toxicity against schizont-infected RBCs. Using this approach we have presented data identifying the first small-molecule inhibitor that blocks malarial parasite entry into RBCs by inhibiting an essential protein–protein interaction. We have demonstrated that the small molecule binds to AMA1 and prevents it from interacting with RON2, resulting in the blockade of a crucial step in invasion, namely, junction formation. In silico docking experiments predict two major ‘hot spot’ regions within the AMA1 hydrophobic pocket that are favourable for inhibitor binding ( Supplementary Fig. S7 ). Although the hydrophobic pocket is the probable binding site of the inhibitors, our data does not rule out the possibility that some of the small molecules may bind outside the pocket and affect the conformation of the hydrophobic pocket. Only a crystal structure can precisely identify the binding site. However, this model provides a starting point for developing the next generation of AMA1–RON2 inhibitors Existing antimalarial drugs primarily target the intracellular stage of the developing parasites. If there are mature parasites that will release merozoites to invade RBCs and sequester despite the presence of drugs in the blood stream [8] , such an added treatment may also reduce disease severity. Resistance to many current antimalarials is primarily due to mutations in either the target protein [36] or a membrane transporter [37] . Resistance to AMA1–RON2 inhibitors is less likely because a single mutation on one of the protein–protein interface may require a complementary mutation in the other to maintain a functional AMA1–RON2 protein complex. This mechanism for inhibition of AMA1–RON2 function holds great promise as a novel therapeutic target. The current AMA1–RON2 inhibitor, although having a low-micromolar IC 50 , provides a proof-of-concept for the identification of more potent inhibitors. More importantly the results presented here highlight the potential for such invasion inhibitors alongside existing antimalarial drugs in the fight against this deadly disease. Protein expression, peptide synthesis and reagents Recombinant, his-tagged AMA1 was made by expressing a codon-optimized AMA1 construct in Pichia pastoris as previously described [38] . Biotin-tagged RON2 peptide (DITQQAKDIGAGPVASCFTTRMSPPQQICLNSVVNTALSTSTQSAMK) with the two cysteines cyclized was synthesized and purified (>95% pure) by LifeTein, LLC USA (New Jersey, USA). AlphaScreen beads including streptavidin-coated donor beads and nickel-coated acceptor beads (catalogue#6760619R) and AlphaScreen biotinylated-(His) 6 control (catalogue#6760303M) were obtained from Perkin-Elmer (Waltham, MA). Source of small-molecule libraries used in this study is shown in Supplementary Fig. S2 . Parasite culture and isolation of invasive merozoites Pf culture-adapted clones (FVO, 3D7, DD2 and HB3) were grown in vitro according to established culture methodologies as described by Trager and Jensen [39] and Haynes et al. [40] Briefly, parasites were grown in RPMI 1640 supplemented with 25 mM HEPES and 50 μg ml −1 hypoxanthine (KD Medical), 0.5% Albumax (Invitrogen), 0.23% sodium bicarbonate (Gibco) using O + RBCs and monitored daily by Geimsa-stained blood smears. Invasive merozoites were isolated from a line of Pf FVO selected for prolonged survival of purified, free merozoites used in a previous study [19] . AMA1–RON2L AlphaScreen assay The AlphaScreen assay was performed according to the manufacturers (Perkin-Elmer) protocol. High-throughput assay development and optimization were carried out in 1,536-well white solid-bottom plates and all incubation steps were carried out at room temperature (RT). A counterscreen assay was performed to identify false-positive compounds that disrupted the energy transfer from donor beads to acceptor beads (quenchers) or ones that nonspecifically disrupted the binding between beads and the linker by substituting a biotinylated-(His) 6 linker for the biotin-RON2L peptide, and his-tagged recombinant AMA1 protein was used. See Supplementary Methods for a detailed description. Coimmunoprecipitation and western blotting Schizont-infected RBCs from synchronized Pf FVO parasites were used for immunoprecipitation. Briefly, 3 × 10 6 schizont-infected RBCs were lysed in the presence of 100 μM of each of the inhibitors in ice-cold parasite-solubilization buffer (50 mM Tris-HCl pH7.5, 150 mM NaCl, 2 mM EDTA, 1% Triton X-100 and protease inhibitor cocktail (Roche). Equal amount of PBS or dimethylsulphoxide (DMSO) was used as a negative control. RON2L peptide (50 μg) that inhibits AMA1–RON complex formation was used as positive control. After incubating on ice for 2 h, samples were centrifuged at 15,000 r.p.m. for 15 min and the supernatant was incubated with mouse anti-RON4 mAb (5 μg). After pulling down the complex using anti-mouse IgG, bound proteins were eluted in SDS loading buffer and run on 5–25% SDS–PAGE gels and transferred to a polyvinylidene difluoride membrane. Blots were probed first with rabbit anti-AMA1 antibody (1:1,000) and detected using horseradish peroxidase (HRP)-conjugated anti-rabbit antibody (1:20,000, Sigma). The same blots were re-probed using mouse anti-RON4 antibody (1:1,000) and detected using conformation-specific HRP-conjugated anti-mouse antibody (eBioscience). Two independent experiments were performed. High-throughput SYBR green assay to measure RBC invasion The assay was performed as described previously [25] with some modifications. Briefly, synchronized schizont-infected RBCs were used for the assay instead of mixed infection, and the assay period was reduced from 72 h to 36 h. See Supplementary Methods for a detailed description. Flow cytometry measurement of merozoite invasion Follow-up assays utilized flow cytometry measurements to evaluate the inhibitory activity of selected compounds. Invasion assays were carried out starting with either purified, schizont-infected RBCs or free, invasive merzoites. For assays using schizont-infected RBCs: fully mature parasites from the FVO, 3D7, DD2 and HB3 clones were purified on a 70–40 percol/sorbitol gradient and mixed with freshly prepared, pre-warmed RBCs. Merozoites were allowed to rupture and invade fresh RBCs (2–4% parasitemia, 1% haematocrit final) for 4–6 h at 37 °C in the presence of varying concentrations of the inhibitors as indicated. For assays using merozoites: merozoites from a Pf clone FVO, selected for prolonged survival were isolated as described previously [19] . Synchronized schizont-infected RBCs were purified on a 70–40 percol/sorbitol gradient and allowed to rupture at 37 °C for 3 h. Merozoites were purified from schizonts by passing twice through a 1.2-micron filter (PALL life sciences). Approximately 5 × 10 7 merozoites were mixed with 2.5 × 10 7 pre-warmed RBCs (500 μl final volume) in the presence of varying concentrations of the inhibitors gassed and incubated at 37 °C for 3–4 h. Free merozoites were removed from RBCs by centrifugation at 50 g for 7 min and the resulting RBC pellet contains newly invaded rings. For flow cytometry measurement, ~5 × 10 7 cells (infected and uninfected RBCs) were incubated with 1X SYBR green (Invitrogen) that labels DNA and mitotracker red (Invitrogen) that stains viable mitochondria for 30 min at RT (final volume 40 μl). Stained cells were diluted by adding 150 μl 1 × PBS. The numbers of ring-infected RBCs were counted using a Accuri C6 flow cytometer (BD biosciences). GraphPad Prism 5.0 software package (San Diego, CA) was used to calculate IC 50 using nonlinear regression. Compound depletion assay His-tagged AMA1 protein (3D7 or FVO allele) or biotin-tagged RON2L peptide (500 pmol each) in 200 μl were captured using dynabeads (Life technologies catalogue # 10103D for His-tagged AMA1 capture or catalogue # 65601 for biotin-tagged RON2L peptide) for 1 h at RT. Unbound protein or peptide was removed and the beads were washed three times with 1 × PBS. Next, the beads were incubated with 500 pmol of the inhibitor (NCGC00262650) in 200 μl and incubated for 1 h at RT. The ability of AMA1- or RON2L-peptide to bind to the inhibitor was tested by capturing the beads on a magnet and collecting the supernatant. Inhibition of merozoite invasion by unbound inhibitor in the supernatants was performed, as described above, using purified, schizont-infected RBCs (FVO clone). Invasion efficiency was measured by counting the number of newly invaded rings by flow cytometry. How to cite this article: Srinivasan, P. et al. Disrupting malaria parasite AMA1–RON2 interaction with a small molecule prevents erythrocyte invasion. Nat. Commun. 4:2261 doi: 10.1038/ncomms3261 (2013).